A violation of the uncertainty principle implies a violation of the second law of thermodynamics Uncertainty relations state that there exist certain incompatible measurements, to which the outcomes cannot be simultaneously predicted. While the exact incompatibility of quantum measurements dictated by such uncertainty relations can be inferred from the mathematical formalism of quantum theory, the question remains whether there is any more fundamental reason for the uncertainty relations to have this exact form. What, if any, would be the operational consequences if we were able to go beyond any of these uncertainty relations? Here we give a strong argument that justifies uncertainty relations in quantum theory by showing that violating them implies that it is also possible to violate the second law of thermodynamics. More precisely, we show that violating the uncertainty relations in quantum mechanics leads to a thermodynamic cycle with positive net work gain, which is very unlikely to exist in nature. Many features commonly associated with quantum physics, such as the uncertainty principle [1] or non-locality [2] , appear highly counter-intuitive at first sight. The fact that quantum mechanics is more non-local than any classical theory [2] , but yet more limited [3] , [4] than what the no-signalling principle alone demands [5] , [6] , [7] has been the subject of much investigation [8] , [9] , [10] , [11] , [12] . Several reasons and principles were put forward that explain the origin of such quantum mechanical limits [10] , [11] , [12] . In ref. 12 , it was shown that the amount of non-locality in quantum mechanics is indeed directly related to another fundamental quantum mechanical limit, namely the uncertainty principle [1] . This forged a relation between two fundamental quantum mechanical concepts. We may however still ask why the uncertainty principle itself is not maybe stronger or weaker than predicted by quantum physics?—and, what would happen if it was? Here we relate this question to the second law of thermodynamics. We show that any violation of uncertainty relations in quantum mechanics (even if the violation is quantitatively small) also leads to a violation of the second law. Fundamental concepts To state our result below, we need to explain three different concepts. First, we need some properties of generalized physical theories (for example, refs 13 , 14 , 15 , 16 , 17 ). Second, we recall the concept of uncertainty relations, and finally the second law of thermodynamics. General theories Although it is not hard to prove our result for quantum theory, we extend our result to some more general physical theories. These are described by a probabilistic framework that makes the minimal assumptions that there are states and measurements, which can be made on a physical system (for example, refs 18 , 19 ). Even for general theories, we denote a state as , where is a convex state space. In quantum mechanics, is simply a density matrix. The assumption that the state space is convex is thereby generally made [17] and says that if we can prepare states and , then the probabilistic mixture prepared by tossing a coin and preparing or with probability each is also an element of . A state is called pure if it cannot be written as a convex combination of other states. Measurements consist of linear functionals called effects. We call an effect pure if it cannot be written as a positive linear combination of any other allowed effects. Intuitively, each effect corresponds to a possible measurement outcome, where is the probability of obtaining ‘outcome’ given the state . More precisely, a measurement is thus given by . For quantum mechanics, we will simply label effects by measurement operators. For example, a projective measurement in the eigenbasis of the Pauli operator is denoted by . The assumption that effects are linear, that is, is linear in , is essentially made for all probabilistic theories [17] and says that when we prepared a probabilistic mixture of states, the distribution of measurement outcomes scales accordingly. Uncertainty relations A modern way of quantifying uncertainty [20] , [21] is by means of entropic uncertainty relations (see ref. 22 for a survey), or the closely related fine-grained uncertainty relations [12] . Here, we will use the latter. As for our cycle, we will only need two measurements with two outcomes, and each measurement is chosen with probability , we state their definition only for this simple case. Let and denote the two measurements with effects and , respectively. A fine-grained uncertainty relation for these measurements is a set of inequalities To see why this quantifies uncertainty, note that if for some , then we have that if the outcome is certain for one of the measurements (for example, ), it is uncertain ( ) for the other. As an example from quantum mechanics, consider measurements in the and eigenbases (we use the common convention of labelling the and eigenbases states as and , respectively). We then have for all pure quantum states The same relation holds for all other pairs of outcomes , and . Depending on , the eigenstates of either or saturate these inequalities. A state that saturates a particular inequality is also called a maximally certain state [12] . For any theory such as the quantum mechanics, in which there is a direct correspondence between states and measurements, uncertainty relations can also be stated in terms of states instead of measurements. More precisely, uncertainty relations can be written in terms of states if pure effects and pure states are dual to each other in the sense that for any pure effect there exists a corresponding pure state , and conversely for every pure state an effect such that . Here, we restrict ourselves to theories that exhibit such a duality. This is often (but not always) assumed [17] , [19] . As a quantum mechanical example, consider the effect and the state . We then have with and . For measurements and consisting of pure effects, let and denote the corresponding dual states. The equation 1 then takes the dual form For our quantum example of measuring in the and eigenbasis, we have , , and . We then have that for all pure quantum effects The same relation holds for all other pairs , and . Again, measurement effects from the eigenstates of either or saturate these inequalities. In analogy, with maximally certain states, we refer to effects that saturate the inequalities (3) as maximally certain effects. From now on, we will always consider uncertainty relations in terms of states. Second law of thermodynamics Finally, the second law of thermodynamics is usually stated in terms of entropies. One way to state it is to say that the entropy of an isolated system cannot decrease. These entropies can be defined for general physical theories, even for systems that are not described by the quantum formalism [19] , [23] , [24] ( Supplementary Methods ). However, for our case, it will be sufficient to consider one operational consequence of the second law of thermodynamics [25] , [26] : there cannot exist a cyclic physical process with a net work gain over the cycle. Main findings Our main result is that if it was possible to violate the fine-grained uncertainty relations as predicted by quantum physics, then we could create a cycle with net work gain. This holds for any two projective measurements with two outcomes on a qubit. By the results of ref. 12 , which showed that the amount of non-locality is solely determined by the uncertainty relations of quantum mechanics and our ability to steer, our result extends to a link between the amount of non-locality and the second law of thermodynamics (note that there is no violation of uncertainty classically, it is rather that classical measurements have at most probabilistic notions of uncertainty to begin with). In the following, we focus on the quantum case, that is, in the situation where all the properties except the uncertainty relations hold as for quantum theory. In the Supplementary Methods , we extend our result to more general physical theories that satisfy certain assumptions. In essence, different forms of entropies coincide in quantum mechanics, but can differ in more general theories [19] , [23] , [24] . This has consequences on whether a net work gain in our cycle is due to a violation of uncertainty alone, or can also be understood as the closely related question of whether certain entropies can differ. Let us now first state our result for quantum mechanics more precisely. We consider the following process as depicted in Fig. 1 . We start with a box, which contains two types of particles described by states and in two separated volumes. The state is the equal mixture of the eigenstates and of two measurements (observables) and . The state is the equal mixture of and . We choose the measurements such that the equal mixture is the completely mixed state in dimension . We then replace the wall separating from by two semi-transparent membranes, that is, membranes which measure any arriving particle in a certain basis and only let it pass for a certain outcome. In the first part of the cycle, we separate the two membranes until they are in equilibrium, which happens when the state everywhere in the box can be described as . Then, in the second part of the cycle, we separate again into its different components. 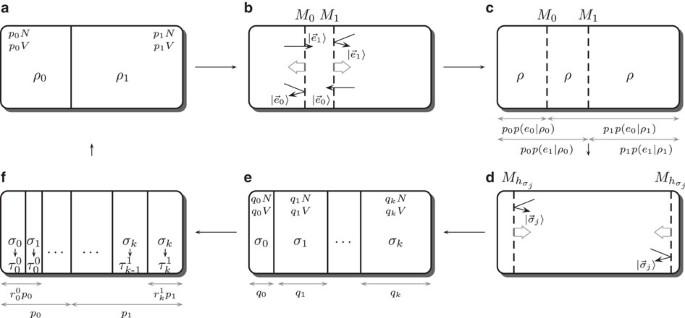Figure 1: The impossible process. At the start (a), two statesρ0andρ1are in separated volumes, containing a total ofNsuch states,N/2 inρ0andN/2 inρ1. Second (b), the wall separating them is replaced by two semi-transparent membranes, of whichM0is transparent for andM1 for . These membranes then move apart until they reach their position at equilibrium (c). This happens when the state in the entire volume can be described by the mixtureρ. New membranes are inserted on the side, and the stateρ=Σjqj|σj〉〈σj| is then (d,e) separated into its pure componentsσjby membranes, which are exactly opaque toσj. In panelf, the volumes are then further subdivided to obtain sizes proportional toand, that is, the weights occuring in the eigen decomposition ofand. We then unitarily transform the pure componentσjin each volume into the corresponding pure componentorofρ0andρ1. Finally, the components ofρ0(ρ1) are mixed to reach the initial configuration (a). Figure 1: The impossible process. At the start ( a ), two states ρ 0 and ρ 1 are in separated volumes, containing a total of N such states, N/ 2 in ρ 0 and N/ 2 in ρ 1 . Second ( b ), the wall separating them is replaced by two semi-transparent membranes, of which M 0 is transparent for and M 1 for . These membranes then move apart until they reach their position at equilibrium ( c ). This happens when the state in the entire volume can be described by the mixture ρ . New membranes are inserted on the side, and the state ρ =Σ j q j |σ j 〉〈 σ j | is then ( d , e ) separated into its pure components σ j by membranes, which are exactly opaque to σ j . In panel f , the volumes are then further subdivided to obtain sizes proportional to and , that is, the weights occuring in the eigen decomposition of and . We then unitarily transform the pure component σ j in each volume into the corresponding pure component or of ρ 0 and ρ 1 . Finally, the components of ρ 0 ( ρ 1 ) are mixed to reach the initial configuration ( a ). Full size image We find that the total work, which can be extracted by performing this cycle is given by Here, is the von Neumann entropy of the state. The entropy appearing in the above expression is simply the Shannon entropy of the distribution over measurement outcomes when measuring in the basis and , respectively (the Shannon entropy of a probability distribution is given by . All logarithms in this paper are to base ). Example To illustrate our result, consider the concrete quantum example, where the states are given by The work that can be extracted from the cycle then becomes The fine-grained uncertainty relations predict in the quantum case that and are at most . We see that a theory, which can violate this uncertainty relation, that is, reach a larger value of , would lead to —a violation of the second law of thermodynamics. We give a strong argument why quantum mechanical uncertainty relations should not be violated. Indeed, as we show, a violation of the uncertainty relations would lead to an ‘impossible machine’, which could extract net work from a cycle. Our result extends to more general theories than quantum theory—however, it raises the question of which general form of entropy [19] , [23] , [24] is most significant. In quantum mechanics, the different entropies of refs 19 , 23 , 24 coincide, meaning that if a physical theory is just like quantum mechanics, but with a different amount of uncertainty, net work can be extracted. We note that of course the quantum mechanical uncertainty relations are a consequence of the mathematical formalism of quantum mechanics. In fact, it is clear from equation 1 that this is the case for all theories. Violating uncertainty relations is thus definitely not consistent with the remainder of a fixed physical theory. Note, however, that the aim of our work is to understand the physical implications of such mathematical boundaries. We show that a violation of uncertainty would have consequences that have a real physical impact on the world around us. Needless to say, ‘breaking’ quantum mechanics in this way may have many other consequences as well—the one demonstrated was simply a rather tangible one. We would like to emphasize that thermodynamical cycles have been useful before to examine foundational questions and our cycle is indeed similar to the ones given in refs 25 , 26 , 27 , 28 . Our contribution lies in the insight that a violation of uncertainty relation allows for the construction of a similar (but not identical) cycle. To explain this relation, let us first consider our result from the perspective of information. We can understand uncertainty relations as given in equation 1 as imposing a limit on how well one of the several bits of information can be extracted from a qubit using the given measurements [12] . As explained in ref. 12 , these uncertainty relation do have an immediate operational interpretation as the average success probability of retrieving individual bits from a bit string, where the average is taken over the choice of bit we want to retrieve. This means that the amount of uncertainty for all pairs of measurements that we could make directly imposes a limit on how much classical information we can store in each qubit. Indeed, in any system that is finite dimensional (possibly due to an energetic constraint), it is thus clear that the mere fact that we can only store a finite amount of information in a finite dimensional system (Holevo's bound [29] ) demands that non-commuting measurements obey uncertainty relations. Otherwise, we could use these measurements to extract more information from the storage system. This shows that our example is closely related to the ones given in refs 26 , 28 , 30 , 31 , where it has been shown that if it was possible to encode more than one bit of information in a qubit and therefore to violate the Holevo bound [29] , then it was also possible to violate the second law of thermodynamics. All these works use a similar cycle than the one proposed in refs 25 , 27 (see also ref. 32 ), which showed that there exists a cycle that leads to an overall net work gain if it was possible to distinguish two non-orthogonal states perfectly. Intuitively, the possibility of distinguishing non-orthogonal states is again directly related to the question of how much information we can store in a quantum state and is thus in spirit similar to the works of refs 26 , 28 , 30 , 31 . Note that for our purpose we need a slightly more refined cycle and analysis, as we do not want to start with an assumption that non-orthogonal states can be distinguished perfectly. Our cycle shows that one does not need to be able to distinguish the non-orthogonal states perfectly, but that a contradiction can be derived as soon as one can distinguish better than allowed by quantum theory. We then forge a quantitative link between the question of how well we can distinguish non-orthogonal states and the violation of uncertainty relations to obtain our result. In future work, it might be interesting to investigate whether an implication also holds in the other direction. Does any violation of the second law lead to a violation of the uncertainty relations? We have investigated the relation between uncertainty and the second law of thermodynamics. A concept related to uncertainty is the one of complementarity. It is an open question, whether a violation of complementarity could also be used to build such an ‘impossible machine’. We now explain in more detail how we obtain the work, which can be extracted from the cycle in quantum mechanics. In the Supplementary Methods , we consider the case of general physical theories. First part of the cycle For the first part of the cycle, we start with two separate parts of the box in each of which there are particles in the states and , respectively. These states are described by where and are chosen such that the state corresponds to the completely mixed state in dimension 2. We then make a projective measurement with two possible outcomes denoted by . More precisely, we insert two semi-transparent membranes instead of the wall separating the two volumes. One of the membranes is transparent to but completely opaque to , while the other lets the particle pass if the outcome is , but not if it was . Letting these membranes move apart until they are in equilibrium, we can extract work from the system. The equilibrium is reached when on both sides of the membrane, which is opaque for , there is the same density of particles in this state and similarly for the membrane, which is opaque for . The work that can be extracted from the first part of the cycle (that is, by going from (a) to (c) in Fig. 1 ) is given by the following ( Supplementary Methods ). where we denoted by the fine-grained uncertainty relations. The inequality can be saturated by choosing and to be maximally certain effects (it is easy to see that in quantum mechanics the maximally certain effects and do indeed form a complete measurement in dimension ). Note that our argument is not specific to the outcome combination and used in the the fine-grained uncertainty relation and choosing the remaining two inequalities corresponding to outcomes and leads to an analogous argument. Example: for our quantum example given by the states (6), we obtain Equality is attained by taking to be the maximally certain effects given by the two eigenstates of . Second part of the cycle In the second part, we form a cycle (that is, we go from (c) to (a) in Fig. 1 via (d) to (f)). We start with the completely mixed state . Denote the different pure components of by , that is, . We can now ‘decompose’ into its components by inserting a semi-transparent membrane, which is opaque for a specific component , but completely transparent for all other components, as depicted in Fig. 1d . Effectively, this membrane measures using the effects that are dual to the states . This membrane is used to confine all states in a volume . This is done for all components and we end up with a box where each component of is sorted in a volume proportional to its weight in the convex combination ( Fig. 1e )). This process needs work proportional to . In a second step (see f) in ( Fig. 1 ), we create the (pure) components of and from the pure components of and then ‘reassamble’ the states and . To do so, we subdivide the volumes containing into smaller volumes, such that the number of particles contained in these smaller volumes are proportional to and . The pure state contained in each small volume is then transformed into the pure state or . As these last states are also pure, no work is needed for this transformation. Finally, we ‘mix’ the different components of together, which allows us to extract work . Similarly, we obtain work from . In total, the transformation , needs work Example: returning to the example above and using that the two eigenvalues of are , we obtain Both and have the two eigenvalues . Therefore, The total work that has to be invested for this process is therefore given by Closing the cycle If we now perform the first and second process described above one after another (that is, we perform a cycle, as depicted in Fig. 1 ), the total work which can be extracted is given by In general, we can see that when the uncertainty relation is violated, this quantity can become positive and a positive corresponds to a violation of the second law of thermodynamics. Example: in our example, the above quantity corresponds to The fine-grained uncertainty relations for quantum mechanics state that . When this value is reached with equality, then in the above calculation. On the other hand, if these values were larger, that is, the uncertainty relation could be violated, then the binary entropy of them would be smaller and becomes positive. How to cite this article: Hänggi, E. & Wehner, S. A violation of the uncertainty principle implies a violation of the second law of thermodynamics. Nat. Commun. 4:1670 doi: 10.1038/ncomms2665 (2013).